New silica clathrate minerals that are isostructural with natural gas hydrates Silica clathrate compounds (clathrasils) and clathrate hydrates are structurally analogous because both materials have framework structures with cage-like voids occupied by guest species. The following three structural types of clathrate hydrates are recognized in nature: cubic structure I (sI); cubic structure II (sII); and hexagonal structure H (sH). In contrast, only one naturally occurring silica clathrate mineral, melanophlogite (sI-type framework), has been found to date. Here, we report the discovery of two new silica clathrate minerals that are isostructural with sII and sH hydrates and contain hydrocarbon gases. Geological and mineralogical observations show that these silica clathrate minerals are traces of low-temperature hydrothermal systems at convergent plate margins, which are the sources of thermogenic natural gas hydrates. Given the widespread occurrence of submarine hydrocarbon seeps, silica clathrate minerals are likely to be found in a wide range of marine sediments. Clathrasils are clathrate compounds of silica with cage-like voids. Clathrasil was first discovered in the form of a rare silica mineral, melanophlogite [1] , [2] , [3] , found in sulphur deposits in Sicily, Italy. Melanophlogite contains various gas molecules such as CH 4 , CO 2 , N 2 and H 2 S in the cage-type pores of the SiO 2 framework [4] , [5] . In the 1980s, three types of clathrasils (melanophlogite [4] , Dodecasil-3C (refs 6 , 7 ) and Dodecasil-1H (ref. 8 )) were successively synthesized. These three clathrasils are isostructural with three types of natural gas hydrates: cubic structure I (sI; 2M 12 ·6M 14 ·46H 2 O), cubic structure II (sII; 16M 12 ·8M 16 ·136H 2 O) and hexagonal structure H (sH; M 18 ·2M 12 ·2M 12 ·34H 2 O), where M X denotes the guest site in the X -faced polyhedral cage. The topologies of these three framework structures are defined by the framework type codes [9] MEP , MTN and DOH , respectively ( Fig. 1 ). 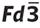Table 1 Summary of the results of Rietveld analyses for chibaite in theandI41/amodels. No description available Figure 1: Framework structures of three types of clathrasils. The framework type codes [9] are ( a ) MEP , ( b ) MTN and ( c ) DOH . The names of silica minerals having these framework types are ( a ) melanophlogite, ( b ) chibaite and ( c ) as yet unnamed. The names of isostructural hydrates are ( a ) structure I (sI), ( b ) structure II (sII) and ( c ) structure H (sH). Full size image Although the structural similarities between clathrasils and clathrate hydrates are well known [3] , [6] , [10] , little is known about potential similarities in their natural occurrences. Melanophlogite has been found at an active submarine vent in the Cascadia margin [11] , where there is a large area of gas hydrate deposits [12] . However, among the three types of clathrasils that are isostructural with natural gas hydrates, only melanophlogite has been found in nature thus far [13] . Although natural gas hydrates occur primarily in the form of sI hydrate [14] , [15] , sII and sH hydrates dominate in some locations [12] , [16] , [17] . The sI hydrate contains mostly biogenic methane, whereas sII and sH hydrates contain larger hydrocarbons in addition to methane [12] , [15] , [17] . These natural gas hydrates occur worldwide in seafloors and permafrost. Because they are one of the largest carbon reservoirs in the shallow geosphere [18] , they have received extensive attention as a potential energy resource, a cause for global climate change [19] and a geological hazard [14] . Interest is also growing in gas hydrates and clathrasils as potential hosts for geological carbon dioxide storage [20] , [21] . The stability fields of sII and sH hydrates are wider than that of sI hydrate, and therefore, the occurrence of sII and sH hydrates is likely an important part of the global distribution of natural gas hydrates [12] . However, details of the carbon cycles in the subsurfaces of these gas hydrates deposits remain poorly understood. Here, we report the discovery of two new silica clathrate minerals that are isostructural with sII and sH hydrates. They were formed in marine sediments at temperatures above stability fields of gas hydrates. We show that the silica clathrate minerals contain hydrocarbon molecules originated from geothermal activities at convergent plate boundary. This occurrence is similar to that of thermogenic gas hydrates in terms of the origin of hydrocarbons and tectonic setting of the occurrence. Silica clathrate minerals store hydrocarbons, which have vanished from sedimentary rocks, and therefore, they provide new evidence about geological carbon cycles at convergent plate boundaries. Locality The silica clathrate minerals were found in marine sediments of Early Miocene age (Hota Group [22] or Emi Group [23] , [24] ) at Arakawa, Minami-boso City, Chiba Prefecture, Japan. The Hota Group is a series of forearc sediments deposited near the plate margin by the Paleo-Izu arc and the triple junction of the Pacific, Philippine Sea and North America plates [23] , [24] . It is composed mainly of tuffaceous siltstone with tuffaceous and volcaniclastic sandstones. They are considered to be the Izu forearc tuffaceous sediments accreted along the proto-Sagami trough during the Early to Middle Miocene subduction of the Philippine Sea plate to Honshu [23] . The silica clathrate minerals occur as veins ranging from a few mm to 1cm thick in tuffaceous sandstone and mudstone of ∼ 18 Ma strata [22] . The sedimentary and deformation structures of the Hota Group show characteristics of the accretionary prism; for example, the web structure, dish structure and hydraulic fracturing structure formed by the removal of high-pressure pore water shortly after sedimentation [23] . These fissures are partly filled with thin veins of calcite, quartz, opal and the silica clathrate minerals. Fine crystals (<1 mm) of pyrite, epistilbite and clinoptilolite have also found in some veins. Minor amount of pyrite is also contained in the sandstone matrix. The matrix pyrite is most probably the source of recrystallized pyrite in veins and fine crystals of gypsum in cracks of sedimentary rocks. Fossils of various shells and carbonized woods have also been found [22] . Optical and physical properties Chibaite is a new mineral analogous to the synthetic MTN -type silica clathrate compound [6] , [7] (approved by the IMA Commission on New Minerals, Nomenclature and Classification: No. 2008-067). The other silica clathrate mineral is as yet unnamed and is analogous to the synthetic DOH -type silica clathrate compound [8] . The euhedral crystals of chibaite are often found in small cavities in veins ( Fig. 2a–c ). Chibaite and the DOH -type mineral are epitaxially intergrown with each other. The <001> axis of the DOH -type mineral is parallel to the <111> axis of chibaite ( Fig. 2d,e ). Chibaite has cubic symmetry with a refractive index of 1.470(1) and a Mohs hardness of 6.5–7. The DOH -type mineral is optically uniaxial and has higher refractive indices than the chibaite. The chibaite crystals often contain domains of low symmetry with anisotropic optical properties. 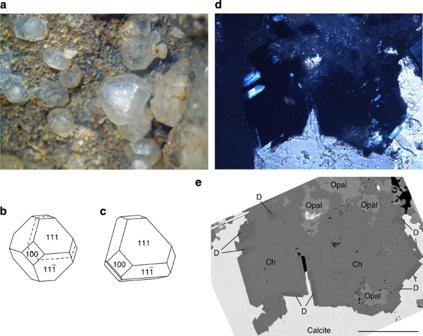Figure 2: Optical and electron probe micro-analyser images of silica clathrate minerals. (a) Euhedral chibaite crystals. Scale bar, 2 mm. (b) Idealized crystal form of a single crystal. (c) Generally observed flattened form of a twinned crystal. (d) Photomicrograph of a thin section under a crossed polarized light. Scale bar, 0.2 mm. (e) Backscattered electron image (BSI) of the thin section. Scale bar, 0.2 mm. TheDOH-type mineral is observed to be slightly darker than chibaite in the BSI image. The optical axis (caxis) of theDOH-type mineral is parallel to the <111> axis of chibaite. Ch: chibaite, D: theDOH-type silica clathrate mineral. Figure 2: Optical and electron probe micro-analyser images of silica clathrate minerals. ( a ) Euhedral chibaite crystals. Scale bar, 2 mm. ( b ) Idealized crystal form of a single crystal. ( c ) Generally observed flattened form of a twinned crystal. ( d ) Photomicrograph of a thin section under a crossed polarized light. Scale bar, 0.2 mm. ( e ) Backscattered electron image (BSI) of the thin section. Scale bar, 0.2 mm. The DOH -type mineral is observed to be slightly darker than chibaite in the BSI image. The optical axis ( c axis) of the DOH -type mineral is parallel to the <111> axis of chibaite. Ch: chibaite, D: the DOH -type silica clathrate mineral. Full size image Chemical composition The chemical analysis of chibaite using an electron probe micro-analyser (EPMA) resulted in the empirical formula Na 0.99 (Si 134.53 Al 1.63 )O 272 , excluding guest gas molecules in the cages. These constituents compose 90–92 wt% (average: 90.89 wt%), and the remaining 8–10 wt% is attributed to the gas molecules. The chemical compositions of optically isotropic and anisotropic chibaite grains do not differ significantly. The hydrocarbons CH 4 , C 2 H 6 , C 3 H 8 and i -C 4 H 10 were detected to be present from the C–C and C–H stretching bands in the Raman spectra ( Fig. 3 and Supplementary Table S1 ). Raman peaks attributable to guest molecules other than hydrocarbons were not detected. Therefore, the ideal formula of chibaite is SiO 2 · n (CH 4 , C 2 H 6 , C 3 H 8 , C 4 H 10 ) with n max =3/17 and Z =136, or Na x (Si 136−x Al x )Σ 136 O 272 ·(CH 4 , C 2 H 6 , C 3 H 8 , C 4 H 10 ) 24−x if Na and Al are considered essential constituents. The calculated density of chibaite is 2.03(1) g cm −3 (see Methods ). The EPMA analysis of the DOH -type mineral gave slightly higher Al contents with 2–3 wt% less total mass than chibaite. 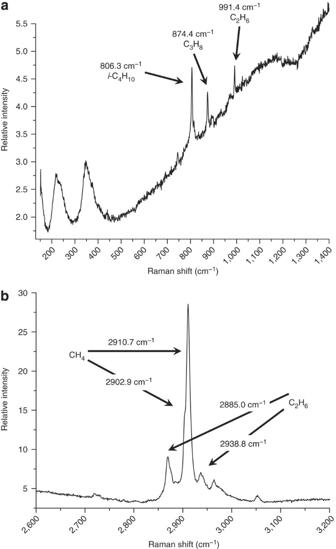Figure 3: Raman spectra of hydrocarbons in chibaite. (a) C–C stretching region. (b) C–H stretching region. The broad Raman peaks lower than 500 cm−1originate from the silica framework structure. SeeSupplementary Table S1for the assignments. Figure 3: Raman spectra of hydrocarbons in chibaite. ( a ) C–C stretching region. ( b ) C–H stretching region. The broad Raman peaks lower than 500 cm −1 originate from the silica framework structure. See Supplementary Table S1 for the assignments. Full size image Crystal structure From the single-crystal X-ray diffraction (XRD) study using a four-circle diffractometer, the lattice parameters of a low-symmetry domain of chibaite in the P 1 setting were refined from 36 strong reflections as a =1.3678(5) nm, b =1.3684(6) nm, c =1.9463(9) nm, α =90.01(4)°, β =89.99(3)° and γ =90.03(3)°, which correspond to a =1.9347 nm and c =1.9463 nm in the setting of the F lattice. However, some of the diffraction peak profiles were split, and the data could not be used for structure determination. Further, single-crystal XRD experiments with a two-dimensional imaging plate detector system suggested that the Laue group of the low-symmetry chibaite is I 4/ m . We also found that only parts of the diffraction spots are split along a certain reciprocal direction. Each individual split spot has a slightly different diffraction 2 θ angle. These observations from optical and XRD studies demonstrate that the cubic and tetragonal domains of chibaite are epitaxially intergrown, and some of the tetragonal domains are most likely oriented with each other according to the relation of pseudo-merohedral twinning. All of the examined samples thus far exhibited a similar nature, and we were not successful in finding a large single crystal suitable for a single-crystal XRD study. The powder XRD data of the sample confirm the existence of both MTN - and DOH -type silica minerals ( Fig. 4 ). When the main diffraction peaks are considered to be those from the cubic chibaite phase with the space group symmetry (ref. 7 ), the unit cell parameters are refined as a =1.93742(3) nm and V =7.2723(2) nm 3 . A small diffraction peak of the 402 reflection was observed ( Supplementary Table S2 ). This peak corresponds to the systematic absence conditions of reflections for the space group and originates from the low-symmetry tetragonal variant of chibaite. The cubic and tetragonal variants of chibaite have the same fundamental structural topologies, and the diffraction peaks from the two phases overlap almost perfectly within the diffractometer resolution. Therefore, an average structure of the cubic and tetragonal chibaite was refined by the Rietveld method [25] . Two structural models with space group symmetry or I 4 1 / a were used because they are reported as space groups of room-temperature phases of MTN -type clathrasil [7] , [26] , [27] . Although there are other possible tetragonal space groups for MTN -type clathrasil [26] , [28] , I 4 1 / a is the highest symmetry space group belonging to the Laue group I 4/ m . The atomic coordinates of quartz and DOH -type mineral phases were not refined, but were fixed at those reported in previous studies because their diffraction peaks are very weak. A brief summary of the Rietveld refinements are listed in Table 1 . The R factors of refinement using the I 4 1 / a model were significantly lower than those obtained using the model. This result suggests that the tetragonal phase is dominant in the examined sample. Rietveld analysis using both the and I 4 1 / a phases as a mixture gave slightly lower R factors ( R wp =4.48%) with fractions of cubic and tetragonal phase at 11 and 79 wt%, respectively. The existence of the tetragonal phase was also clarified by powder XRD data of another sample measured under higher resolution conditions ( Fig. 5 ). Details of the crystallographic study are disclosed in the Methods and Supplementary Table S3 . Structure parameters for chibaite in the I 4 1 / a model and for the DOH -type mineral are listed in Supplementary Tables S4 and S5 . 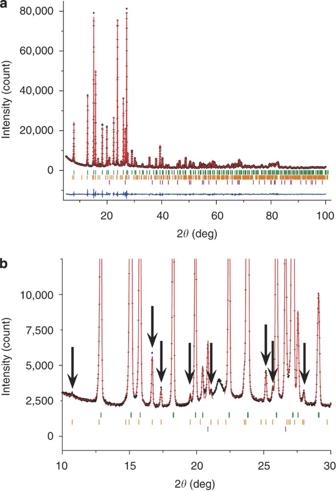Figure 4: Observed (cross), calculated (red line) and difference (blue line) XRD patterns for the Rietveld refinement of the sample. (a) The entire region. (b) Enlarged view of low-angle part. The tick marks represent the calculated peak positions for chibaite (green), theDOH-type mineral (orange) and quartz (purple), in descending order. The arrows inbshow diffraction peaks from theDOH-type mineral. Figure 4: Observed (cross), calculated (red line) and difference (blue line) XRD patterns for the Rietveld refinement of the sample. ( a ) The entire region. ( b ) Enlarged view of low-angle part. The tick marks represent the calculated peak positions for chibaite (green), the DOH -type mineral (orange) and quartz (purple), in descending order. The arrows in b show diffraction peaks from the DOH -type mineral. Full size image Table 1 Summary of the results of Rietveld analyses for chibaite in the and I 4 1 / a models. 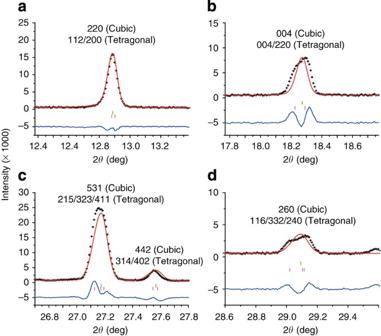Figure 5: Powder XRD peak profiles of chibaite measured at a high-resolution setting. Observed (black cross), calculated (red line) and difference (blue line) profiles at 2θrages of (a) 12.38–13.38°, (b) 17.77–18.77°, (c) 26.7–27.8° and (d) 28.6–29.6°. The calculated profiles are the result of Le Bail fitting in the 2θrange from 6.5 to 31.1° using a cubic unit cell. The tick marks represent the calculated peak positions of the cubic (green) and tetragonal (pink) chibaite phases. The splitting of the cubic 004 and 260 reflections into the tetragonal 004/220 reflections and 116/332/240 reflections, respectively, are observed. Shifts of the peak positions from those of the ideal cubic phase and irregular variations of peak widths also show the presence of the tetragonal phase. Full size table Figure 5: Powder XRD peak profiles of chibaite measured at a high-resolution setting. Observed (black cross), calculated (red line) and difference (blue line) profiles at 2 θ rages of ( a ) 12.38–13.38°, ( b ) 17.77–18.77°, ( c ) 26.7–27.8° and ( d ) 28.6–29.6°. The calculated profiles are the result of Le Bail fitting in the 2 θ range from 6.5 to 31.1° using a cubic unit cell. The tick marks represent the calculated peak positions of the cubic (green) and tetragonal (pink) chibaite phases. The splitting of the cubic 004 and 260 reflections into the tetragonal 004/220 reflections and 116/332/240 reflections, respectively, are observed. Shifts of the peak positions from those of the ideal cubic phase and irregular variations of peak widths also show the presence of the tetragonal phase. Full size image The space group symmetries of some clathrasils are known to be dependent on temperature and pressure. At high temperatures, the space groups of melanophlogite and MTN -type clathrasil have the highest symmetries of n and m , respectively [29] , [30] . They undergo symmetry-lowering on distortion of the frameworks with a decrease in temperature or an increase in pressure [26] , [29] , [31] . In contrast, the cubic and tetragonal chibaite phases coexist at the same temperature and pressure. This coexistence most likely reflects variations in the guest molecules in chibaite, as the space group symmetry of MTN -type clathrasil is also dependent on guest molecules [26] and chibaite contains various hydrocarbons at least up to C≤4. The coexistence of DOH -type mineral with chibaite indicates that there were even larger hydrocarbons at the time of their crystallization because DOH -type clathrasil crystallizes when there are large guest molecules that cannot be incorporated into the MTN -type framework [32] . In addition to chibaite and the DOH -type mineral, we found indirect evidence for the coincidental occurrence of melanophlogite, although melanophlogite itself has yet to be discovered in the same place. This indirect evidence is the presence of two types of quartz pseudomorphs after clathrasils; that is, crystals that were initially grown as clathrasil, but were transformed into polycrystalline quartz while preserving their original external shapes during subsequent diagenesis. The first type is a white pseudomorph after chibaite. This pseudomorph preserves the hexagonal platy shape of chibaite. The other type is a cubic-shaped translucent pseudomorph ( Supplementary Fig. S1 ), which must have initially grown as melanophlogite because melanophlogite is the only silica mineral with a cubic crystal habit. Quartz pseudomorphs after melanophlogite are also common in other melanophlogite localities [2] . These observations demonstrate that all three types of clathrasils that are isostructural with sI, sII and sH gas hydrates occur under certain environments in marine sediments. Hydrocarbon gases in marine sediments originate from two sources: biogenic and thermogenic sources. The biogenic hydrocarbons consist of more than 99.9% methane [33] , and they form sI-type methane hydrate [15] . This microbial methane in sI hydrate had migrated a short distance or had been generated by in-situ methanogenesis [15] . In contrast, hydrocarbons larger than ethane are characteristic of thermogenic hydrocarbons, and they form sII- and sH-type hydrates [12] , [17] . Thermogenic hydrocarbons are generated by the decomposition of organic matter deep below the seafloor at temperatures above ∼ 100 °C (refs 34 , 35 ), and they migrate to the seafloor through faults and mud volcanoes [36] , [37] . Chibaite and the DOH -type mineral contain various hydrocarbons, such as methane, ethane, propane and isobutane. This hydrocarbon composition suggests that the source of hydrocarbons in these minerals was thermogenic. At the locality of the present study, fossils of chemosynthetic shells such as Calyptogena sp., Acharax tokunagai , Conchocele bisecta and Lucinoma acutilineata have been found [22] . These chemosynthetic communities demonstrate the presence of hydrocarbon gas seeps that are often associated with gas hydrate deposits [38] , [39] . No evidence has been found for the presence of volcanic hydrothermal systems in the Hota group because this area was far away from the volcanic front at the time of sedimentation. The Hota group in the Arakawa area is in fault-contact with ophiolitic rocks of the Mineoka belt. These ophiolitic rocks intruded into the Hota group shortly after the sedimentation of the Hota group. These geological structures indicate that this area has been adjacent to the plate boundary. In addition to various deformation structures, the strata of the Hota group at another location contain blocks, veins and pipes of calcic concretions, which are similar to those observed in other subduction zones [23] . Some of these calcic concretions contain blocks of accidental rocks, indicating diapiric intrusions of deeper sediments into the Hota group. The δ 13 C value with respect to the PeeDee Belemnite standard is a major indicator of the source of CO 2 in carbonates: seawater of 18 Ma= ∼ +1 to +2‰ (ref. 40 ), magmatic= ∼ −3 to −7‰ (ref. 41 ). Microbial methanogenesis by the reduction of CO 2 is the source of the lightest methane (δ 13 C<−60‰) and is accompanied by residual CO 2 enriched for δ 13 C. The δ 13 C values of carbonates associated with shallow gas hydrate deposits and gas seeps are often reported to be very small ( ∼ −20 to −50‰), because the oxidation of isotopically light methane is the main source of CO 2 in these carbonates [39] , [42] . In contrast, the carbon isotope ratio of calcite associated with chibaite is found to be relatively 13 C-enriched, at +3.5±0.2‰. This value could be due to the alteration of marine carbonates or the mixing of pyrolytic CO 2 ( ∼ −20‰) with 13 C-enriched CO 2 . However, the alteration of marine carbonates is less likely because the host rocks are tuffaceous and rarely contain carbonate minerals, except for the calcic concretions of diapiric blocks and veins. Furthermore, 13 C-enriched CO 2 (δ 13 C>+5‰) is generated by isotopic fractionation in mud volcanoes by secondary methanogenesis following anaerobic biodegradation of thermogenic hydrocarbons [43] , [44] . This origin of CO 2 is consistent with the thermogenic character of the gas composition of chibaite. The formation depth and temperature of the silica clathrate minerals can be estimated from the association with opal-A. During the diagenetic processes, opal-A transforms into opal-CT and then opal-CT transforms into quartz. The transformation proceeds through the dissolution and precipitation of silica minerals because of differences in their solubility. Opal-A converts almost completely to opal-CT when burial temperatures reach approximately 35–50 °C, and quartz forms extensively when temperatures reach ∼ 80 °C (refs 45 , 46 ). Opal-CT has been argued to form at much lower temperatures, at least as low as 17–21 °C (ref. 47 ). Because silica clathrate minerals are closely associated with opal-A and are rarely in contact with quartz, they could be formed at burial depths shallower than approximately 1.5–3 km at temperatures at least as low as 50–80 °C. The most important pathway for migration of deeply buried hydrocarbons to the seafloor is mud volcanoes, which are the geological structures formed as a result of the emission of unlithified sediments from at least deeper than 1–1.5 km [37] . They are also one of the significant sources of atmospheric methane [37] . The driving forces for such diapiric migrations of argillaceous materials and fluids are mainly gravitational instability and pore-fluid pressure caused by rapid sedimentation rates and tectonic stress or expansion [36] , [37] . Therefore, mud volcanoes are situated in active areas of plate boundaries and in zones of young orogenic structures. Thermogenic gas hydrate deposits are abundantly distributed in these active areas in association with faults and mud volcanoes [36] ; for example, the Gulf of Mexico [16] , [17] , [39] , the Cascadia margin [12] , [38] , the Black Sea [42] , the Barbados accretionary prism [34] , the Costa Rica forearc [48] , the Gulf of Cadiz [35] and the Mediterranean Sea [49] . Accordingly, hydrocarbons contained in thermogenic gas hydrates and those contained in chibaite and DOH -type mineral are of the common origin, which is the thermal decomposition of organic matter in deep sediments. There are common features in the geological and tectonic settings of their occurrences. The difference is the formation temperature: gas hydrates occur in cold environments near the seafloor, whereas silica clathrate minerals occur in deeper and warmer areas. The thermodynamic stabilities of various clathrasils are not measurably different from each other [13] , [50] . Therefore, the variety of silica clathrate minerals reflects the variety of gas molecules in natural environments as template molecules. Our findings show that the formation of the sedimentary structure of the Hota group involved the release of a substantial amount of thermogenic hydrocarbons during the formation of accretionary prism. Given the widespread occurrence of thermogenic hydrocarbon gas seeps at active plate boundaries, silica clathrate minerals are likely to be found as a common host for hydrocarbons in these areas. Because the presence of silica clathrate minerals serves as direct evidence for vanished hydrocarbons in sedimentary rocks, they provide a new means for understanding the geological carbon cycle from dewatered ancient mud volcanoes. Chemical analysis The chemical analyses were performed using the electron probe micro-analyser JEOL JXA-8800M (WDS mode, 15 kV, 10 nA, 1-μm beam diameter, JEOL). The Raman spectra of chibaite were measured using a JASCO NRS-2000 (JASCO). The hydrocarbon contents were not determined directly because of the small amounts of material available. The density calculation was based on the chemical composition Na 1.00 (Si 134.52 Al 1.64 )O 272 ·15.0(CH 4 )·8.0(C 4 H 10 ), where the amounts of hydrocarbons were assumed based on the crystal structure: (Na+CH 4 )=16 atoms per formula unit (a.p.f.u.) and C 4 H 10 =8 a.p.f.u. Carbon isotope measurement The carbon isotope ratio of calcite was measured by an elemental analyser (Carlo Erba, EA1108) connected to an isotope ratio mass spectrometer (Finnigan Mat, MAT 252). The measurability of the carbon isotope ratio with EA-irMS was checked in previous studies [51] and in this study. The complete decomposition of calcite under the present analytical conditions was checked with in-house standards (calcite and an organic compound). The accuracies of the carbon isotope ratios were also checked with the in-house calcite standard (+5.5‰). XRD study Single-crystal XRD studies were performed using an automated four-circle diffractometer (MacScience, MXC3) and an imaging plate diffractometer (Rigaku, R-AXIS IV++). The powder XRD (PXRD) data were collected using a powder diffractometer (Bruker AXS, D8-Advance Vario-1) in a modified Debye–Scherrer geometry using Cu K α 1 radiation from a primary monochromator. A high-speed 1D-PSD detector (Bruker AXS, VÅNTEC-1, detection 2 θ angle of 12.9°) was used at step intervals of 0.017438° and 42 s per step. The powder sample was prepared from several grains of nearly pure chibaite crystals up to 1 mm in size, which were carefully separated from the host rock under an optical microscope. A borosilicate capillary tube with an inner diameter of 1.0 mm was used, and the capillary specimen was spun during the measurement. The most high-resolution PXRD data for Figure 5 were collected on the above diffractometer with measurement conditions as follows: a narrow detection angle of 6°, soller slits of narrow aperture angle (1°) and a thin capillary tube with an inner diameter of 0.5 mm. The obtained diffraction data were analysed by the Rietveld method using a programme RIETAN-FP [52] . The split pseudo-Voigt function of Toraya was used as a profile function, and a partial profile relaxation was applied to isolated reflections in the low 2 θ region. The initial structure parameters of the framework of chibaite and DOH -type mineral were taken from those reported for Dodecasil-3C 7 and Dodecasil-1H 8 . The I 4 1 / a model of chibaite was generated from the model by using VESTA [53] . The Si–O bond lengths and Si–O–Si bond angles were restrained within 0.160±0.002 nm and 109.47±2.0°, respectively. The atomic coordinates of quartz and DOH -type mineral were not refined, but were fixed at those reported in previous studies. Coordinates of guest molecules in chibaite were refined by trial and error. Coordinates of guest molecules in DOH -type mineral were fixed at peak positions in the difference Fourier maps in the previous study [8] . Sample The type specimen of chibaite was deposited in the Tohoku University Museum (Mineral collection A-151). How to cite this article: Momma, K. et al . New silica clathrate minerals that are isostructural with natural gas hydrates. Nat. Commun. 2:196 doi: 10.1038/ncomms1196 (2011).